Transcriptional refractoriness is dependent on core promoter architecture Genes are often transcribed in random bursts followed by long periods of inactivity. Here we employ the light-activatable white collar complex (WCC) of Neurospora to study the transcriptional bursting with a population approach. Activation of WCC by a light pulse triggers a synchronized wave of transcription from the frequency promoter followed by an extended period ( ∼ 1 h) during which the promoter is refractory towards restimulation. When challenged by a second light pulse, the newly activated WCC binds to refractory promoters and has the potential to recruit RNA polymerase II (Pol II). However, accumulation of Pol II and phosphorylation of its C-terminal domain repeats at serine 5 are impaired. Our results suggest that refractory promoters carry a physical memory of their recent transcription history. Genome-wide analysis of light-induced transcription suggests that refractoriness is rather widespread and a property of promoter architecture. mRNA transcripts are often present at only a few copies per cell [1] , [2] , [3] . Yet, transcription of genes appears to be a smooth process when analysed in an ensemble of cells. However, analyses of transcriptional dynamics of single genes in single cells have revealed that transcription is often highly unstable and discontinuous [4] , [5] , [6] . Thus, many genes are transcribed in bursts, with brief periods of high activity (gene ‘on’) interspersed by long periods of inactivity (gene ‘off’). Burst size, that is, the number of transcripts per burst, and burst frequency, that is, the number of transcriptional bursts per time unit are gene specific and appear to depend on the promoter architecture, such as the presence of a CAAT box, a TATA box, the size of the nucleosome-free region as well as the location and number of transcription factor binding sites [7] , [8] , [9] , [10] , [11] , [12] . Burst sizes of between 1 and >50 transcripts per burst have been observed followed by periods of inactivity of up to several hours [7] , [8] , [12] , [13] , [14] , [15] , [16] , [17] , [18] , [19] . Stochastic processes (noise) of unknown origin contribute to the temporal variability of transcription within one cell and between cells [15] , [20] , [21] . However, the duration of the periods of transcriptional inactivity may not be entirely stochastic. Rather, recent evidence suggests that processes associated with transcription itself appear to induce extended time periods during which genes are refractory towards activation [12] , [22] , [23] . Molecular mechanisms underlying such refractoriness of promoters are not known. By analysing burst statistics under distinct experimental regimes, single-cell-based studies provide valuable insight into the dynamics of transcription. However, they are generally not suited for unravelling underlying biochemical processes, as conventional biochemical measurements are usually performed on an ensemble of cells and cannot readily be applied to single cells. Since transcriptional bursts of identical promoters in a population are not correlated in steady state, a population-based analysis requires tight synchronization of cells by rapid induction of transcription in the entire population, which can be conceptualized as a superposition of the transcriptional dynamic of many individual cells. More importantly, biochemical characterization of the refractory period that may follow a transcriptional burst requires a synchronized challenge of the ensemble of refractory promoters. The kinetics of application, but particularly of withdrawal and reapplication, of conventional biochemical transcription inducers is generally too slow to allow a time-resolved analysis of a synchronized population of cells. Here we describe and characterize a natural light-inducible gene expression system based on the transcription activator and blue-light photoreceptor White collar complex (WCC) of Neurospora crassa (for review see refs 24 , 25 ). The system allows repetitive stimulation of transcription within a short period of time. We show that activation of the WCC by a single short light pulse (LP) triggers a synchronized wave of transcription at a large number of promoters. A detailed time-resolved biochemical analysis of the light-inducible frequency ( frq ) promoter revealed that the activated promoter becomes refractory towards further stimulation for about 1 h. We show that refractoriness is independent of the previously reported frq antisense transcript that has been suggested to interfere with frq sense transcription [26] and mechanistically distinct from photoadaptation mediated by the blue-light photoreceptor VVD [27] . When challenged during the refractory period the frq promoter efficiently recruits WCC. The recruited WCC is fully active and has the potential to interact with Pol II to activate transcription. However, recruitment of Pol II and phosphorylation of serine 5 of its heptade C-terminal domain repeats is compromised, suggesting that the refractory promoters are blocked. Genome-wide analysis indicates that many light-inducible promoters become refractory after activation and suggests that the extent of refractoriness is a promoter-specific feature. Light-induced synchronization of frq and vvd transcription A number of features suggested that the light-activatable transcription factor WCC of Neurospora and the frequency ( frq ) promoter are suitable for studying biochemical processes associated with transcriptional bursting in a synchronized population approach ( Supplementary Fig. 1a,b ). (i) In darkness frq is rhythmically transcribed at low levels under control of WCC that binds to the clock-box located ∼ 1.2 kb upstream of the transcription start site [28] . Light rapidly activates WCC by triggering a stable FAD-cysteinyl photoadduct [29] , [30] . (ii) Light, in contrast to conventional chemical inducers, can be administered instantly at any concentration (intensity) and the inducer can be withdrawn immediately by switching lights off. Hence, it should be possible to titrate the fraction of activated WCC in vivo . (iii) The light-activated WCC is rapidly inactivated by phosphorylation [27] , [31] , [32] . In constant light the activity of the WCC is additionally attenuated by the small photoreceptor VVD, a process termed photoadaptation [27] , [31] , [32] ( Supplementary Fig. 2 ). (iiii) Activated WCC binds to a light-responsive element (LRE) and fully activates the frq promoter at low light intensity [27] . It should therefore be possible to repeatedly challenge the frq promoter under functionally saturating conditions by activating portions of the WCC with consecutive LPs. We tested these hypotheses: When dark grown Neurospora was exposed to a 1-min high-LP (50 μmol photons m −2 s −1 ) the WCC was transiently phosphorylated ( Fig. 1a ). Phosphorylation, which is detected by a change in electrophoretic mobility of WC1, is indicative of deactivation of the WCC [31] . Phosphorylation was detected 15 min after the LP and increased progressively for at least 30 min. Time-resolved RNA-seq indicates that the transiently active WCC induced synchronized waves of transcription at the frq and vvd loci. The transcripts accumulated in the course of 15 min and were then rapidly degraded ( Fig. 1b,c ). 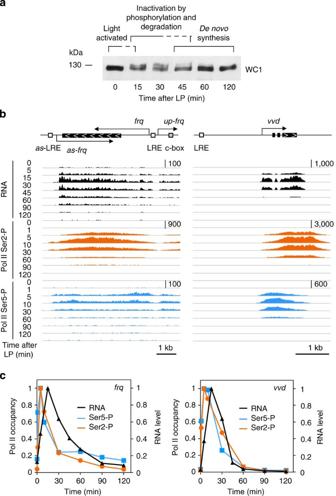Figure 1: Light-induced synchronized transcription wave at thefrqandvvdpromoters. Neurosporawas exposed to a 1-min saturating LP (50 μmol m−2s−1) and analysed after the indicated time periods. (a) Transient phosphorylation of WC1 in response to the LP. The phosphorylation state of the WC1 subunit in response to the 1 min LP was analysed after the indicated time periods by western blot. (b) The rapid activation and inactivation kinetics of the WCC drives synchronized waves of transcription from thefrqandvvdpromoters. Thefrqandvvdloci are schematically outlined (top). ORFs are represented by black boxes with white chevrons. Thefrqclock-box (C-box) and light-responsive elements (LRE) offrqandvvdare indicated. Arrows indicate sense (frq), antisense (as-frq) and upstream (up-frq) transcripts as well as thevvdtranscript. The approximate transcription start sites (TSSs) were estimated from RNA-seq and Pol II Ser5-P ChIP-seq profiles. Time-resolved RNA-seq and ChIP-seq of Pol II Ser5-P and Ser2-P in response to the LP were visualized with IGV genome browser. (c) Temporal profiles of Pol II Ser5-P (blue) and Pol II Ser2-P (orange) occupancy and accumulation of transcript level (black) atfrq(left panel) andvvd(right panel). Data from (b) were quantified and maxima were set to 1. Figure 1: Light-induced synchronized transcription wave at the frq and vvd promoters. Neurospora was exposed to a 1-min saturating LP (50 μmol m −2 s −1 ) and analysed after the indicated time periods. ( a ) Transient phosphorylation of WC1 in response to the LP. The phosphorylation state of the WC1 subunit in response to the 1 min LP was analysed after the indicated time periods by western blot. ( b ) The rapid activation and inactivation kinetics of the WCC drives synchronized waves of transcription from the frq and vvd promoters. The frq and vvd loci are schematically outlined (top). ORFs are represented by black boxes with white chevrons. The frq clock-box (C-box) and light-responsive elements (LRE) of frq and vvd are indicated. Arrows indicate sense ( frq ), antisense ( as-frq ) and upstream ( up-frq ) transcripts as well as the vvd transcript. The approximate transcription start sites (TSSs) were estimated from RNA-seq and Pol II Ser5-P ChIP-seq profiles. Time-resolved RNA-seq and ChIP-seq of Pol II Ser5-P and Ser2-P in response to the LP were visualized with IGV genome browser. ( c ) Temporal profiles of Pol II Ser5-P (blue) and Pol II Ser2-P (orange) occupancy and accumulation of transcript level (black) at frq (left panel) and vvd (right panel). Data from ( b ) were quantified and maxima were set to 1. Full size image Phosphorylation of the C-terminal domain heptameric repeats of RNA polymerase II at serine 5 (Pol II Ser5-P) and serine 2 (Pol II Ser2-P) is indicative of transcription initiation and transcription elongation/termination [33] , [34] , respectively. ChIP-seq analysis with specific antibodies ( Supplementary Fig. 3 ) of the temporal occupancy profiles of Pol II Ser5-P and Ser2-P indicated that the LP induced a tightly synchronized wave of frq transcription that peaked after ∼ 5 min and then abated ( t ½ ∼ 20 min) rapidly ( Fig. 1b,c ). Comparable results were obtained by ChIP–qPCR ( Supplementary Fig. 4a ). Analysis of the temporal profiles of the initiating Pol II Ser5-P ( Fig. 1b ) and strand-specific analysis of frq transcripts ( Supplementary Fig. 4b ) revealed that transcription initiation from sense and antisense frq promoters is equally efficient. The wave of transcription from the vvd promoter was ∼ 10-fold higher than from the frq promoter ( Fig. 1b ), indicating that the vvd promoter is stronger. The LP induced similarly confined transcription waves from other light-induced genes ( Supplementary Fig. 4c ). Interestingly, RNA-seq and Pol II ChIP-seq analysis revealed that the frq light-responsive element (LRE) controls in addition to frq RNA also a divergently (in upstream direction) transcribed RNA ( up-frq ) of unknown function ( Fig. 1b , left). Titration of the WCC with light The light-induced formation of a stable covalent photoadduct ( t ½ ∼ 4 h) in the LOV domain [27] , [30] acts on an individual WCC like a digital switch. Hence, exposure to a non-saturating LP should separate the ensemble of WCCs into two distinct pools, an irreversibly activated and a non-activated dormant fraction. When Neurospora was exposed to LPs of increasing intensity the phosphorylation state of the WCC pool increased ( Fig. 2a and Supplementary Fig. 5a ), indicating that the fraction of activated WCC can indeed be titrated in vivo with LPs of different intensity. To measure the response of frq and vvd promoters to LPs of increasing intensity we used luciferase ( luc ) reporter genes ( Supplementary Fig. 5b ). To facilitate quantification of the LP-induced transcription waves we chose a stable luciferase ( t ½ ∼ 6–8 h) [35] . Luciferase levels accumulated for ∼ 1 h after the LP and then decreased rather slowly ( Supplementary Fig. 5c ). Since the turnover of luc RNA is much faster than the turnover of luciferase [35] , the maximal luciferase levels ( ∼ 1–2 h after the LP) are approximately proportional to a temporal integration of the number of mRNA molecules produced in response to the LP irrespective of the shape (peak heights versus width) of the transcription wave. As expected, vvd – luc was expressed at higher levels than frq – luc ( Supplementary Fig. 5c ). Expression levels of frq – luc saturated with LPs of low intensity ( ∼ 1 μmol m −2 s −1 ), that is, with a low fraction of activated WCC, while vvd – luc levels reached saturation at a photon concentration of ∼ 20 μmol m −2 s −1 ( Fig. 2b and Supplementary Fig. 5c ). Quantification by qRT–PCR of the endogenous frq and vvd RNA yielded similar results for the saturating light intensities ( Fig. 2c ). 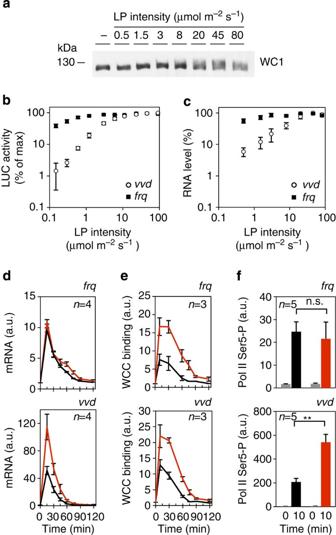Figure 2: Titration of the WCC with light. (a) Controlled activation of fractions of the WCC by titration with light. The phosphorylation state of the WC1 subunit in response to a 1 min LP of the indicated intensity is shown. Samples were collected 30 min after the light pulse and WC1 was analysed by western blot. (b,c) Differential saturation offrqandvvdpromoters by the light-activated WCC. (b) Strains expressing single genomic copies offrq–lucandvvd–lucreporter genes were exposed to a 1-min LP of the indicated intensity. Luciferase activity was determinedin vivo90 min after the LP (±s.e.m.;n=3). Maximalfrq–lucandvvd–luclevels were normalized to 100%. (c)Neurosporawas exposed to 1 min LPs of the indicated intensity. Samples were collected after 15 min andfrqandvvdRNA was quantified by qRT–PCR. Maximal levels offrqandvvdRNA were normalized to 100% (±s.e.m.;n=3). (d–f) Light-dependent recruitment of WCC and Pol II Ser5-P tofrqandvvd. Mycelia were exposed to a 2 μmol m−2s−1low LP (black lines and bars) or a 50 μmol m−2s−1high LP (red lines and bars) and analysed after the indicated time periods. (d) qRT–PCR offrqandvvdRNA. ChIP–qPCR of (e) WC2 and (f) Pol II Ser5-P. (±s.e.m.,n=3 to 5; n.s.: not significant; **P<0.005, unpaired two-tailedt-test). Figure 2: Titration of the WCC with light. ( a ) Controlled activation of fractions of the WCC by titration with light. The phosphorylation state of the WC1 subunit in response to a 1 min LP of the indicated intensity is shown. Samples were collected 30 min after the light pulse and WC1 was analysed by western blot. ( b , c ) Differential saturation of frq and vvd promoters by the light-activated WCC. ( b ) Strains expressing single genomic copies of frq–luc and vvd–luc reporter genes were exposed to a 1-min LP of the indicated intensity. Luciferase activity was determined in vivo 90 min after the LP (±s.e.m. ; n =3). Maximal frq–luc and vvd–luc levels were normalized to 100%. ( c ) Neurospora was exposed to 1 min LPs of the indicated intensity. Samples were collected after 15 min and frq and vvd RNA was quantified by qRT–PCR. Maximal levels of frq and vvd RNA were normalized to 100% (±s.e.m. ; n =3). ( d – f ) Light-dependent recruitment of WCC and Pol II Ser5-P to frq and vvd . Mycelia were exposed to a 2 μmol m −2 s −1 low LP (black lines and bars) or a 50 μmol m −2 s −1 high LP (red lines and bars) and analysed after the indicated time periods. (d) qRT–PCR of frq and vvd RNA. ChIP–qPCR of ( e ) WC2 and ( f ) Pol II Ser5-P. (±s.e.m., n =3 to 5; n.s. : not significant; ** P <0.005, unpaired two-tailed t- test). Full size image Next, we quantified frq and vvd RNA as well as recruitment of WCC and Pol II in response to a low LP (2 μmol m −2 s −1 ) and a high LP (50 μmol m −2 s −1 ). As expected, the amount of frq RNA was independent of the intensity of the LP while the vvd promoter did not saturate at low-LP intensity. The induced level of vvd RNA was much higher than the frq RNA level ( Figs 2d and 1b ). Despite the huge difference in transcriptional output, recruitment of WCC to frq and vvd LREs was comparable and at both promoters dependent on the intensity of the LP ( Fig. 2e ). This apparent discrepancy between transcriptional output and binding site occupancy is due to the ChIP procedure. ChIP analysis corresponds to a time- and population-averaged occupancy of binding sites since only a fraction of binding events is generally captured by FA-crosslinking [36] , [37] , [38] , [39] . Hence, quantification of ChIP does not allow distinguishing between stable binding of transcription factors to only a fraction of promoters in the population versus dynamic binding/unbinding of transcription factors to all promoters for only a fraction of the time (cross-linking period). Since WCC-induced transcription at the frq promoter saturated at low-LP intensity, each (activatable) promoter in the population must have recruited at least one molecule of WCC. If the WCC were stably bound the ChIP efficiency at the frq LRE should be maximal (saturated) at low-LP intensity, which was not the case. Hence, the dependence of WCC occupancy (ChIP) on LP intensity indicates that the WCC is not stably bound but equilibrates (that is, rapidly binds and unbinds) on the timescale of the cross-linking period ( Supplementary Fig. 6 ). Apparently, a fraction of the WCC binding/unbinding events induced by the high-intensity LP was sufficient to trigger the maximal transcriptional output of the frq promoter. Additional binding/unbinding events occur and are detected by ChIP but are functionally futile. In contrast, the time averaged WCC occupancy of the vvd LRE correlated well with the magnitude of the transcriptional output of the vvd promoter. We noticed that WCC occupancy (dynamic binding/unbinding) of both promoters persisted longer ( t ½ ∼ 60 min) than the corresponding transcript levels (t ½ ∼ 30 min), indicating that the transcription factor (which is phosphorylated at that time, see Fig. 1a ) and/or the promoters were inactivated in response to the LP. The amount of initiating Pol II (Pol II Ser5-P) at the frq and vvd promoters ( Fig. 2f ) correlated with the levels of frq and vvd RNA, respectively, but not with binding of the WCC to these promoters. Thus, Pol II Ser5-P occupancy was independent of LP intensity at the frq promoter and dependent on LP intensity at the vvd promoter. Furthermore, significantly more Pol II was recruited to the vvd promoter ( Fig. 2f ). Altogether the data suggest that light-induced transcription at the frq promoter is limited at the level of transcription initiation. In contrast, transcription initiation is fast and efficient at the vvd promoter such that the (dynamic) WCC occupancy level correlates with the rate-limiting step of transcription under the conditions investigated. The frq promoter is refractory towards restimulation Since the frq promoter can be saturated by activation of a small fraction of WCC, it should be possible to subsequently challenge the promoter by activating additional, dormant WCC with a second LP. Under the same experimental regime the WCC-dependent transcriptional output of the vvd promoter can be used as a measure to estimate the fraction of activated WCC. We exposed frq – luc and vvd – luc initially to a 2 μmol m −2 s −1 low LP ( Fig. 3a ), which was saturating for the frq promoter but activated only a fraction of the WCC (<50%, see Fig. 2a–c ). The mycelia were subsequently challenged with a high LP to activate the remaining dormant WCC. The frq promoter barely responded to a challenging high-LPs administered 15 min after the low LP ( Fig. 3a , upper panel). The response was half maximal to a LP given 60 min after the first LP and maximal after ∼ 2 h ( Fig. 3a , middle and lower panels). Quantification of corresponding analyses indicated that activation of the frq promoter by the first LP rendered the promoter refractory to subsequent restimulation for a time period of t ½ ∼ 1 h ( Fig. 3b ). Challenging frq – luc with two consecutive low LPs yielded corresponding results ( Supplementary Fig. 7 ). The vvd promoter was not saturated by the low LP and responded to subsequent high LPs ( Fig. 3c ), confirming that refractoriness of the frq promoter was not caused by limiting WCC levels. 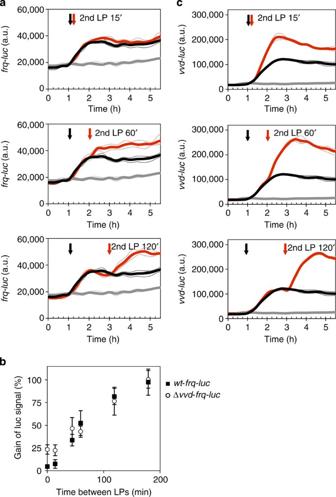Figure 3: Previously activatedfrqpromoters are refractory to restimulation. (a) Mycelial cultures offrq–lucwere incubated in a 96-well format in the dark and luciferase activity was continuously recorded (grey traces). After 1-h cultures were exposed to a low LP (2 μmol m−2s−1; black arrows and traces) or to a low LP and subsequently challenged with a high-LP (50 μmol m−2s−1, red traces) at the indicated time points (red arrows) and luciferase activity was continuously recorded. Thick traces correspond to the average luciferase activity of three individual cultures (thin traces). (b) Transcription of thefrqpromoter induces a refractory period of∼60 min. WT (black squares) and Δvvd(white circles) mycelial cultures offrq–lucreceived a 1-min saturating low LP (2 μmol m−2s−1) and then a second high-LP (50 μmol m−2s−1) 0, 15, 45, 60, 120 or 180 min after the first LP. The gain of luciferase signal relative to the first LP was determined. (±s.e.m.,n=3). (c) Mycelial cultures ofvvd–luc were analysed as described in (a). Figure 3: Previously activated frq promoters are refractory to restimulation. ( a ) Mycelial cultures of frq – luc were incubated in a 96-well format in the dark and luciferase activity was continuously recorded (grey traces). After 1-h cultures were exposed to a low LP (2 μmol m −2 s −1 ; black arrows and traces) or to a low LP and subsequently challenged with a high-LP (50 μmol m −2 s −1 , red traces) at the indicated time points (red arrows) and luciferase activity was continuously recorded. Thick traces correspond to the average luciferase activity of three individual cultures (thin traces). ( b ) Transcription of the frq promoter induces a refractory period of ∼ 60 min. WT (black squares) and Δ vvd (white circles) mycelial cultures of frq – luc received a 1-min saturating low LP (2 μmol m −2 s −1 ) and then a second high-LP (50 μmol m −2 s −1 ) 0, 15, 45, 60, 120 or 180 min after the first LP. The gain of luciferase signal relative to the first LP was determined. (±s.e.m., n =3). ( c ) Mycelial cultures of vvd –luc were analysed as described in ( a ). Full size image The vvd gene encodes a LOV-domain photoreceptor that is required for photoadaptation of transcription in constant light (see Supplementary Fig. 2b ). To analyse whether the refractory behaviour of the frq promoter is affected by VVD and related to photoadaptation, we measured the response to LPs of frq – luc in a Δvvd strain. The frq promoter was also refractory in the absence of VVD ( Fig. 3b ) demonstrating that refractoriness is functionally distinct from VVD-mediated photoadaptation. Biochemical characterization of refractory promoters We then biochemically characterized refractory frq promoters when challenged with a second LP ( Fig. 4 ). To induce the refractory state mycelia were exposed to a low LP that activated sufficient WCC to functionally saturate the frq promoter. As expected, frq RNA levels were rapidly induced in response to the LP and decreased after 15 min ( Fig. 4a , upper panel). After 30 min the mycelia were then exposed to a high-LP to activate the pool of dormant WCC. The response of the frq promoter to the second LP was attenuated ( ∼ 1/3 of the initial response), confirming that 30 min after the first LP most of the frq promoters were still refractory. We followed binding of the WCC by ChIP–qPCR ( Fig. 4b , upper panel). WCC was recruited after the first LP and the occupancy of the frq promoter decreased slightly after 15 min. In response to the subsequent high LP the WCC was more efficiently recruited to the frq promoter. The increased (time averaged) occupancy correlated with the elevated level of WCC activated by the high-LP but not with the transcriptional output of the frq promoter, indicating that newly activated WCC binds efficiently to refractory frq promoters and equilibrates rapidly with the (old) WCC activated by the previous low LP. 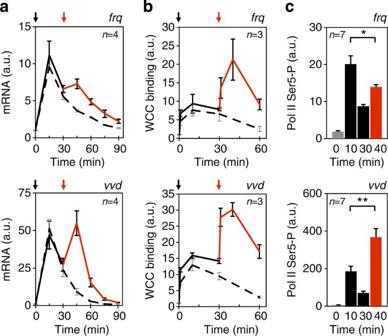Figure 4: Refractoryfrqpromoters recruit newly activated WCC but transcription initiation is blocked. Neurosporawas exposed to a low LP (black arrows) and challenged after 30 min by a high-LP (red arrows) andfrqandvvdgenes were analysed (upper and lower panels, respectively). (a) Samples were collected after the indicated time periods andfrqandvvdRNA was quantified by qRT–PCR. Levels offrqandvvdRNA before the light pulse were set to 1. Control cells received only the first low LP (dotted black lines). In parallel samples were cross-linked (10 min) with formaldehyde (FA) and subjected to ChIP with antibodies against WC2 (b) and Pol II Ser5-P (c). Precipitated DNA was quantified by qRT–PCR for enrichment of thefrqandvvdLRE (WC2) and thefrqandvvdTSS (Pol II Ser5-P), respectively. Error bars represent ±s.e.m. (n=3–7; *P<0.05,**P<0.005, unpaired two-tailedt-test). Figure 4: Refractory frq promoters recruit newly activated WCC but transcription initiation is blocked. Neurospora was exposed to a low LP (black arrows) and challenged after 30 min by a high-LP (red arrows) and frq and vvd genes were analysed (upper and lower panels, respectively). ( a ) Samples were collected after the indicated time periods and frq and vvd RNA was quantified by qRT–PCR. Levels of frq and vvd RNA before the light pulse were set to 1. Control cells received only the first low LP (dotted black lines). In parallel samples were cross-linked (10 min) with formaldehyde (FA) and subjected to ChIP with antibodies against WC2 ( b ) and Pol II Ser5-P ( c ). Precipitated DNA was quantified by qRT–PCR for enrichment of the frq and vvd LRE (WC2) and the frq and vvd TSS (Pol II Ser5-P), respectively. Error bars represent ±s.e.m. ( n =3–7; * P <0.05,** P <0.005, unpaired two-tailed t- test). Full size image We then asked whether Pol II was recruited to the refractory promoters ( Fig. 4c , upper panel). Pol II Ser5-P was transiently detected after the first LP, while the signal was significantly lower after the second LP, that is, the Pol II recruitment dynamics was similar to the frq RNA profile. Corresponding results were obtained for the frq – luc reporter gene ( Supplementary Fig. 8 ), excluding a potential contribution of frq antisense ( as-frq ) transcription (see Fig. 1b ). In contrast, vvd RNA levels as well as WCC binding and Pol II Ser5-P occupancy of the vvd promoter increased in response to the second LP, confirming that the vvd promoter was not functionally saturated after the initial low LP ( Fig. 4a–c , lower panels). To obtain a spatiotemporal resolution of Pol II occupancy dynamics we followed Pol II transcription in response to consecutive low and high LPs by ChIP-seq analysis of Pol II Ser5-P (initiating), Pol II Ser2-P (elongating) and total Pol II. The Pol II occupancy profiles at the frq and vvd loci ( Fig. 5a ) confirmed that the frq promoter was refractory towards restimulation. The low abundance of Pol II before the challenging high LP suggests that refractory frq promoters and transcription units were not blocked by stalled Pol II. However, while transcription initiation in response to the challenging LP was compromised in the direction of frq transcription the spatial resolution of the Pol II ChIP-seq analysis revealed that the WCC recruited to the frq LRE was obviously interacting with Pol II to initiate expression of the divergently transcribed up-frq RNA ( Fig. 5a,b ). This demonstrates that active WCC was recruited to the frq LRE in response to the second LP. We found five more examples of divergently oriented light-inducible transcripts ( Supplementary Fig. 9 ). At least at three of these loci the divergent promoters appeared to respond differentially to the challenging high LP. The data suggest that refractoriness is promoter specific. 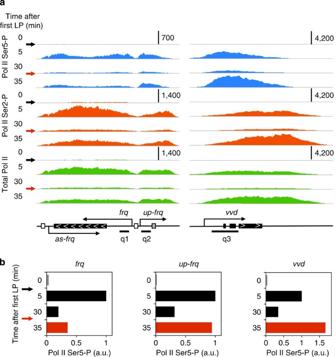Figure 5: Differential transcription dynamics of the divergentfrqandup-frqpromoters controlled by a common LRE. Mycelial cultures were exposed to a low LP (black arrows) and challenged after 30 min by a high LP (red arrows). At the indicated times samples were subjected to FA cross-linking (10 min) and ChIP-seq with Pol II antibodies. (a) Temporal profiles of Pol II Ser5-P (blue), Pol II Ser2-P (orange) and total Pol II (green) occupancy atfrq(left panel) andvvd(right panel) loci. Bottom: schematic representation offrqandvvdgenes and transcripts (seeFig. 1b). q1, q2 and q3 indicate 0.5-kb regions used to quantify Pol II Ser5-P occupancy offrq,up-frqandvvdpromoters, respectively. (b) Quantification of the temporal profile of Pol II Ser5-P occupancy atfrq,up-frqandvvdpromoters. Pol II Ser5-P ChIP-seq reads 5 min after the low LP were set to 1. Figure 5: Differential transcription dynamics of the divergent frq and up-frq promoters controlled by a common LRE. Mycelial cultures were exposed to a low LP (black arrows) and challenged after 30 min by a high LP (red arrows). At the indicated times samples were subjected to FA cross-linking (10 min) and ChIP-seq with Pol II antibodies. ( a ) Temporal profiles of Pol II Ser5-P (blue), Pol II Ser2-P (orange) and total Pol II (green) occupancy at frq (left panel) and vvd (right panel) loci. Bottom: schematic representation of frq and vvd genes and transcripts (see Fig. 1b ). q1, q2 and q3 indicate 0.5-kb regions used to quantify Pol II Ser5-P occupancy of frq , up-frq and vvd promoters, respectively. ( b ) Quantification of the temporal profile of Pol II Ser5-P occupancy at frq , up-frq and vvd promoters. Pol II Ser5-P ChIP-seq reads 5 min after the low LP were set to 1. Full size image To assess whether the up - frq promoter, the c-box or the frq LRE affect the refractory behaviour of the frq promoter we either deleted the region upstream of the frq LRE or replaced the LRE of the frq promoter by the LRE of vvd ( Fig. 6a ). The frq promoters fused to a luciferase-PEST reporter were, like the frq promoter, saturated by low-intensity LPs ( Supplementary Fig. 10 ). We then measured LUC PEST expression of frqΔup-luc PEST and frq-vvdLRE-luc PEST in response to consecutive low and high LPs. The chimeric promoters were refractory towards restimulation ( Fig. 6b ) indicating that the core frq promoter (−67 bp to +153 bp) holds the information for refractoriness. 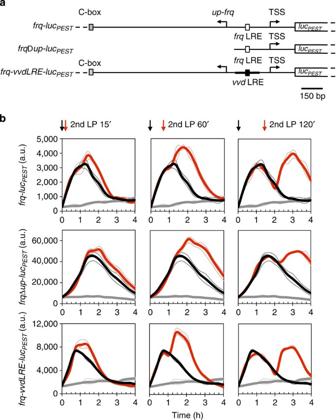Figure 6: Refractoriness is associated with the corefrqpromoter. (a) Schematic offrqpromoter versions. Thefrqpromoter (2,720 bp; top), a truncated version lacking theup-frqpromoter (379 bp; middle) and a chimericfrqpromoter with thevvdLRE (2,726 bp; bottom) were fused to a luciferase gene encoding a PEST-destabilised protein (lucPEST). The constructs were integrated into the genome at thehis3locus of abdstrain. (b) Mycelial cultures of the indicated strains were incubated in the dark (grey traces) or exposed to a low LP (2 μmol m−2s−1; black arrows and traces) or to a low LP and subsequently challenged with a high-LP (50 μmol m−2s−1, red traces) at the indicated time points (red arrows). LUCPESTactivity was continuously recorded. Thick traces correspond to the average luciferase activity of three individual cultures (thin traces). Figure 6: Refractoriness is associated with the core frq promoter. ( a ) Schematic of frq promoter versions. The frq promoter (2,720 bp; top), a truncated version lacking the up-frq promoter (379 bp; middle) and a chimeric frq promoter with the vvd LRE (2,726 bp; bottom) were fused to a luciferase gene encoding a PEST-destabilised protein ( luc PEST ). The constructs were integrated into the genome at the his3 locus of a bd strain. ( b ) Mycelial cultures of the indicated strains were incubated in the dark (grey traces) or exposed to a low LP (2 μmol m −2 s −1 ; black arrows and traces) or to a low LP and subsequently challenged with a high-LP (50 μmol m −2 s −1 , red traces) at the indicated time points (red arrows). LUC PEST activity was continuously recorded. Thick traces correspond to the average luciferase activity of three individual cultures (thin traces). Full size image The data indicate that refractory behaviour is a feature of previously activated frq promoters. Refractoriness is neither associated with the frq upstream transcript nor with the frq LRE. Furthermore refractoriness is not affected by the noncoding frq antisense RNA (not present in the luc reporter genes). Since all reporter constructs were integrated into the his-3 locus, refractoriness of the frq promoter is neither associated with genomic localization (that is, endogenous frq and frq in his3 locus are refractory) nor with global or local availability of active WCC (that is, frq and vvd behave differently in the same genomic locus). The extent of refractoriness is promoter specific On a genome-wide scale we identified 71 promoters that were transiently and rapidly induced to a substantial extent (more than twofold) by the initial low LP. Hence, these promoters are likely direct targets of the WCC. The transcriptional activity of these promoters (Pol II occupancy) in response to the challenging high LP varied over a broad range ( Fig. 7a and Supplementary Fig. 11 ). The transcriptional activity of about half of the promoters was attenuated, indicating that these promoters were refractory towards restimulation. The other promoters, which responded stronger to the high-LP, are either not refractory or refractory to a low extent or short time period. Examples of the dynamics of Pol II Ser5-P occupancy are shown for the strongly refractory non-anchored cell wall protein-6 promoter and the potentially non-refractory albino 1 promoter ( Fig. 7b left and middle panels). The refractory and non-refractory transcription dynamics of these promoters was confirmed by quantification of the respective transcripts by qRT–PCR ( Fig. 7b , right panels). Further examples are shown in Supplementary Fig. 12 . 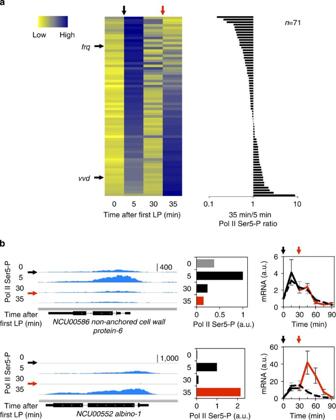Figure 7: Genome-wide identification of refractory light-inducible promoters. Mycelial cultures were exposed to a low LP (black arrows) and challenged after 30 min by a high-LP (red arrows). After the indicated time periods samples were subjected to FA cross-linking and ChIP-seq with Pol II Ser5-P antibodies. (a) Left panel: heat map of temporal Pol II Ser5-P profiles of 71 highly light-inducible genes (see Methods section). Data are sorted in ascending order according to the 35 min/5 min Pol II Ser5-P ratio. Right panel: promoter refractoriness plot. The ratios of Pol II Ser5-P occupancy 5 min after the challenging high-LP versus the Pol II Ser5-P occupancy in response to the initial low LP are shown for the 71 light-inducible promoters. (b) Temporal profiles of Pol II Ser5-P (left and middle panels) are shown for the highly refractory non-anchored cell wall protein-6 promoter and the (apparently) non-refractoryalbino 1promoter. Right panel: quantification of corresponding transcript levels by qRT–PCR. (±s.e.m.,n=4). Figure 7: Genome-wide identification of refractory light-inducible promoters. Mycelial cultures were exposed to a low LP (black arrows) and challenged after 30 min by a high-LP (red arrows). After the indicated time periods samples were subjected to FA cross-linking and ChIP-seq with Pol II Ser5-P antibodies. ( a ) Left panel: heat map of temporal Pol II Ser5-P profiles of 71 highly light-inducible genes (see Methods section). Data are sorted in ascending order according to the 35 min/5 min Pol II Ser5-P ratio. Right panel: promoter refractoriness plot. The ratios of Pol II Ser5-P occupancy 5 min after the challenging high-LP versus the Pol II Ser5-P occupancy in response to the initial low LP are shown for the 71 light-inducible promoters. ( b ) Temporal profiles of Pol II Ser5-P (left and middle panels) are shown for the highly refractory non-anchored cell wall protein-6 promoter and the (apparently) non-refractory albino 1 promoter. Right panel: quantification of corresponding transcript levels by qRT–PCR. (±s.e.m., n =4). Full size image Altogether the data suggest that refractoriness of light-inducible promoters is rather common. The extent of refractoriness varies over a broad range and seems to be dependent on promoter sequence or architecture. We present a population approach for the biochemical analysis of refractory promoters that complements recent statistical analyses of transcription dynamics in single cells [12] , [23] , [40] . Our assay is based on rapid and tight synchronization of transcription by the light-inducible transcription factor WCC of Neurospora . This system allows activation and restimulation of promoters by quantized and time restricted activation of sub-fractions of the WCC with LPs of different intensity and subsequent time-resolved analysis of the synchronized promoter population by conventional bulk biochemical methods such as ChIP-seq. The WCC is a natural photoreceptor and transcription factor and we study natural light-inducible promoters under physiologically relevant conditions. A number of powerful optogenetic gene expression systems with genetically engineered light-inducible [41] , [42] , [43] , [44] or even light-switchable transcription factors [45] have been developed in the recent years. Such systems are used with great success for localized induction of genes but may in principle also be suited for the study of refractoriness of promoters with biochemical means in population-based approaches similar to the one described here. However, since transcription is a combinatorial process of considerable complexity a natural system might be more suitable. Thus, recruitment of a TF and activation of transcription is often facilitated by other TFs and generally induces a complex series of events, including recruitment of coactivators, chromatin modifiers and remodelers, general TFs and Pol II [46] , [47] , [48] . Some genetically engineered TFs with simple activation domains such as VP16 motifs [44] , [49] may not fulfil all these functions in a fully efficient manner and may thus not trigger sufficiently synchronized waves of transcription in an ensemble of cells. Furthermore, inducible promoters often contain tandem arrays of TF-binding sites [44] , [49] and it is not known whether the chromatin context of such artificial promoters is physiological. Whether natural promoter systems with (bio)chemical inducers may also be suitable for the biochemical analysis of transcriptional refractoriness will depend on the dynamics of repetitive induction of transcription waves. We show here that frq promoters, when induced by the light-activated WCC, become refractory towards restimulation. Refractoriness is immediately induced and, hence, does not require light-induced synthesis and accumulation of a putative inhibitor. When refractory frq promoters are challenged with newly activated WCC, the transcription factor readily binds to LREs of the refractory promoters and exchanges with the previously activated (old) WCC. The newly recruited WCC recruits Pol II, which initiates transcription in the up-frq direction. Recruitment of Pol II and transcription initiation in the frq direction is, however, attenuated during the refractory period. The up-frq promoter does, however, not affect the refractory behaviour of the frq promoter. Similarly, the frq antisense promoter has no effect on refractoriness since it is not present in the frq – luc reporter genes. Our ChIP analyses of WCC and Pol II indicate that refractory frq promoters are neither physically blocked by a previously deactivated transcription factor nor blocked by a stalled Pol II complex. Rather, the data suggest that the frq promoter region is modified or remodelled during the preceding transcription burst, creating a rather inactive state that must be reversed to reactivate the promoter. Such potential modification/remodelling is promoter specific and could be triggered by deactivated WCC that dynamically interacts with refractory promoters for a prolonged time period or by components of the general transcription machinery. Nucleosomes are an obvious target for cis-acting processes [50] , [51] associated with transcriptional refractoriness, but coactivators such as Mediator and SAGA or general transcription components of the preinitiation complex could also be targets [34] , [52] , [53] , [54] , [55] , [56] , [57] . In particular, after the transcribing Pol II has left the transcription start site, a scaffold composed of Mediator, TFIID, TFIIA, TFIIH and TFIIE remains at the promoter, which can recruit new Pol II to form a reinitiation complex [58] . Modification of components of this platform could interfere with efficient transcription reinitiation. The directed generation of selective tools will help analysing whether a platform of modified transcription machinery remains associated with refractory promoters. Transcriptional bursting and probably also refractoriness seem to be rather widespread but are probably not ubiquitous [11] , [12] , [22] , [23] . The transient blockage of transcription initiation observed at refractory frq promoter may not be the only mechanism governing refractory transcription dynamics. In particular, genome-wide constraints that modulate transcriptional kinetics could also result in transcriptional bursting and refractoriness [11] , [18] , [59] . Furthermore, it has recently been shown that limiting topoisomerase causes transcriptional bursting in bacteria since transcription-induced torsional stress in DNA is not efficiently relaxed [60] . Torsional stress induced by limited topoisomerase may not be responsible for the long refractory periods characterized here, since refractoriness is promoter-specific even in an identical genomic location. Yet, like in bacteria, refractoriness could represent an off-pathway reaction that could be viewed as transcription-induced stress. In this case, machinery must exist that removes the off-pathway products to maintain transcriptional homeostasis [61] . Alternatively, transcriptional bursts and the subsequent refractory period may represent sequential on-pathway intermediates triggered by maturation of transcription factors and/or the local transcription machinery. Since accumulation of a gene product in response to a transcriptional stimulus takes quite some time, quantized transcription pulses interrupted by long refractory periods may set windows of opportunity for the accumulation of gene products and their appropriate feedback on promoter activity. Transcriptional bursting may thus prevent potentially harmful overexpression of induced genes. In this case, machinery may exist that modulates gene expression on the level of transcription burst size and burst frequency [7] , [11] , [14] , [18] , [61] , [62] . The WCC system described here provides a powerful tool for time-resolved biochemical analysis of refractory promoters and associated machinery. Strains and culture conditions Strains indicated with bd carry the ras-1 bd mutation [63] . Fungal Genetics Stock Center (FGSC) #2489 was used as the wild-type strain for RNA-seq and ChIP-seq experiments. Standard growth medium contained 2% glucose, 0.5% L -arginine, 1 × Vogel’s medium. If not indicated otherwise, cells were grown 36 h in constant light (LL) and 24 h in constant darkness (DD) before the specific light treatment. Plasmid construction and Neurospora transformation Construction of the vector containing frq-vvdLRE - luc PEST was performed in three steps. A pFH62-luc PEST plasmid [35] was used as parental plasmid. An AscI and a XbaI sites were introduced by site-directed mutagenesis up- and downstream, respectively, of the frq LRE. A 151-bp fragment containing the vvd LRE was amplified by PCR and inserted into the AscI and XbaI sites. frq ▵ up luc PEST was constructed by inserting a 387-bp synthetic frq promoter fragment into the BamH1 and NotI sites of pFH62-luc PEST . The synthetic promoter contains a SphI and a Asc1 site 107 bp upstream and 153 bp downstream of the TSS (+1), respectively. Luc reporters and luc PEST reporter genes were inserted into the his-3 locus of the indicated bd strains. Primers are listed in Supplementary Table 1 and the frq ▵ up sequence in Supplementary Table 2 . RNA analysis RNA was prepared with peqGOLD TriFAST (PeqLab). The reverse transcription was done with the QuantiTect reverse transcription kit (Qiagen) following the manufacturer’s instructions. Strand-specific cDNA for actin , frq and frq antisense RNA were amplified with specific primers as described [64] . Transcript levels were analysed by quantitative real-time PCR in 96-well plates with the StepOnePlus real-time PCR system (Applied Biosystems). TaqMan Gene Expression Master Mix (Applied Biosystems), TaqMan, and UPL probes (Roche) were used. Primers and probes are listed in Supplementary Table 3 . Antibodies Polyclonal anti-rabbit antibodies were raised and purified using standard techniques. Pol II Ser2-P was raised against the peptide (pS)PTSPSY(pS)PTSPS C , Pol II Ser5-P against SPT(pS)PSYSPT(pS)PS C and Pol II total against the N-terminal sequence YFAHSSAPLRTIKEIQS C . WC2 antibodies were raised against a GST-WC-2 protein expressed in Escherichia coli [65] . WC1 rabbit antibodies were raised against the C-terminal peptide C REEMGEHQQGLSV and affinity purified. The cysteinyl residues ( C ) were added to allow coupling of the peptides to SulfoLink coupling resin for affinity purification of antibodies. Chromatin immunoprecipitation (ChIP) ChIP was performed as described previously [66] . Four hundre microlitres grounded mycelia was sonicated using a Covaris S220X sonicator (180 peak power, 20.0 duty factor, 200 cycles/bursts, for 4 min at 4 °C). Total extracts were subjected to ChIP with specific affinity purified antibodies with ( ∼ 1 μg antibody). Primers and probes used for the ChIP–qPCR are listed in Supplementary Table 3 . In vivo luciferase measurements Light-pulse assay: standard growth medium contained 2% glucose, 0.5% L -arginine, 1 × Vogel’s and 150 μM firefly luciferin. Ninety-six-well plates were inoculated with 1.5 × 10 5 conidia per well and incubated in darkness for 20 h at 25 °C. Plates were then exposed to the indicated light pulse regime. Bioluminescence was recorded in darkness at 25 °C with an EnVision Xcite Multilabel Reader. Protein analysis Neurospora protein extraction was performed as described [32] . Protein concentration was estimated by measuring absorption at 280 nm (NanoDrop, PeqLab). Western blotting was performed as described [67] . Nitrocellulose filters were stained with Ponceau S to control uniform loading of the gels. Antibodies against WC1 were used 1:500 diluted in 5% milk, Pol II Ser2-P antibodies at a dilution of 1:2,000 and Pol II Ser5-P antibodies at a dilution of 1:1,000 in 5% milk. Enhanced chemiluminescence signals were detected with X-ray films. Uncropped scans of the western blots are shown in Figure Supplementary Fig 13 . RNA and ChIP sequencing cDNA was prepared with NEBNext Ultra RNA Prep kit and NEBNext Multiplex oligos. ChIP DNA libraries were prepared with NEBNext ChIP-Seq Library Prep Reagent Set for Illumina with NEBNext Multiplex oligos. A 2100 Bioanalyser was used for quality control of libraries. Fifty base pairs unpaired sequencing was performed with a HiSeq 2000 at GeneCore EMBL Heidelberg. High-throughput data analysis Raw reads were mapped to Neurospora crassa genome (NC10) using Bowtie [68] . Three mismatches were allowed and reads mapping to more than one location were discarded. RNA-seq analysis: Gene expression was quantified by counting reads falling into exons. Normalization was carried out using the size factor formula as described [69] . Pol II (Ser2-P, Ser5-P and Total) ChIP-seq analysis: The median of Pol II reads in extragenic regions was used for normalization. If not stated otherwise Pol II occupancy was quantified by the number of reads falling into a 500 bp window centred around the stop codon (Pol II Ser2-P) and the start codon (Pol II Ser5-P) and by the number of reads falling into annotated ORFs (total Pol II). Normalized gene expression is shown in Supplementary Tables 4–6 . Pol II Ser5-P ChIP-seq was used to identify light-induced genes. Differentially expressed genes were determined as fold change>2 compared with dark reads and P <0.05. Genes showing a maximal Pol II Ser5-P occupancy 5 min after LP were defined as direct light-induced genes. Accession codes: RNA and ChIP sequencing data have been deposited in the GenBank sequence read archive (SRA) under the accession codes SRR1538715 to SRR1538717 . How to cite this article: Cesbron, F. et al. Transcriptional refractoriness is dependent on core promoter architecture. Nat. Commun. 6:6753 doi: 10.1038/ncomms7753 (2015).